A synthetic route to ultralight hierarchically micro/mesoporous Al(III)-carboxylate metal-organic aerogels Developing a synthetic methodology for the fabrication of hierarchically porous metal-organic monoliths that feature high surface area, low density and tunable porosity is imperative for mass transfer applications, including bulky molecule capture, heterogeneous catalysis and drug delivery. Here we report a versatile and facile synthetic route towards ultralight micro/mesoporous metal-organic aerogels based on the two-step gelation of metal-organic framework nanoparticles. Heating represents a key factor in the control of gelation versus crystallization of Al(III)-multicarboxylate systems. The porosity of the resulting metal-organic aerogels can be readily tuned, leading to the formation of well-ordered intraparticle micropores and aerogel-specific interparticle mesopores, thereby integrating the merits of both crystalline metal-organic frameworks and light aerogels. The hierarchical micro/mesoporosity of the Al-metal-organic aerogels is thoroughly evaluated by N 2 sorption. The good accessibility of the micro/mesopores is verified by vapour/dye uptake, and their potential for utilization as effective fibre-coating absorbents is tested in solid-phase microextraction analyses. Metal-organic frameworks (MOFs) [1] that consist of metal ions/clusters and organic struts have been widely investigated as a new class of porous solids and have promising applications in gas storage, separation, catalysis and drug delivery [2] , [3] , [4] . One advantage of crystalline MOFs is the regular array of well-defined pores, which can achieve ultrahigh porosity and surface area [5] , [6] . Nevertheless, their pore sizes are typically restricted to the microporous regime (<2 nm). The synthesis of mesoporous MOFs (pore size>2 nm) is expected to enhance the diffusion capability of the channels while facilitating practical applications that require bulky molecules transportation [7] , [8] , [9] , [10] , [11] . Recently, preparations of MOFs that incorporate micro/mesoporosities have been attempted under the aid of surfactants [12] , [13] or by mechanochemistry [14] ; even so, other obstacles, such as the production and immobilization of MOFs in an easy-handling shape or monolith, remain with respect to their industrial use [15] , [16] , [17] . Aerogels are known to possess versatile porosity, low density and high internal surface area properties. Moreover, this type of porous material can easily be used to make monolithic solids of desired shapes and is proven to work for applications such as heterogeneous catalysis, adsorption/separation technology and membrane/film processing [18] , [19] . Unfortunately, the design of the aerogel is still rudimentary owing to a large disorder present in the structure and the insufficient prediction of gelation behaviour [20] . Nevertheless, metal coordination is emerging as an effective force when used to drive gelation, offering metal-organic gels (MOGs) as a novel class of functional soft materials [21] , [22] , [23] in which the scaffolding framework is fabricated by metal–ligand coordination in conjunction with other supramolecular interactions (for example, hydrogen bonding, π-π stacking). Considering the inherent correlation between MOFs and MOGs with comparable bonding connectivity but different structural regularity, a promising approach to generating a meso/macroporous gel matrix by utilizing microporous MOF particles (MOFPs) as the building units is expectable. On the other hand, various functional materials based on nanoscale metal-organic particles (NMOPs) have already been documented [4] , [24] , [25] , [26] . Recently, thixotropic metallogels derived from NMOPs of 1D coordination chains [27] and a colloidal route to the preparation of optical thin films of nanoporous MOFs [28] were reported. These works may shed light on the design of MOGs based on crystalline nano-MOFPs; further, it is of interest to produce hierarchically porous metal-organic aerogels (MOAs) at relatively low cost with readily handled shapes that can combine the ordered microporosity of MOFs with the significant accessibility of MOGs. Therefore, the gelation behaviour of MOFPs deserves systematic exploration that is reminiscent of the occasional observations of gel formation in common MOF syntheses. Here, in an effort to establish a viable gelation process based on nanosized MOFP subunits containing well-defined microporosity, we report a general synthetic route for the fabrication of low density and highly porous MOA materials via MOG formation from the stepwise assembly of light metal Al(III) with bridging carboxylic acids ( Fig. 1 ). Such porous solids may derive their merits from both MOFs and MOGs by (1) bridging the gap between MOFs and MOGs to achieve hierarchical micro- and mesoporosity, (2) putting the local order of nanoscale MOFPs into an amorphous gel matrix to enable structural tuning and growth control, (3) enhancing the pore accessibility of MOFs to open doors for more practical purposes and (4) making such syntheses and applications more readily processed. 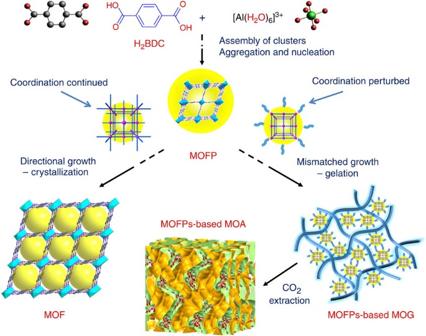Figure 1: Schematic representation of the formation of MIL-53(Al) MOF versus AlBDC MOA. MOF, metal-organic framework; MOFP, metal-organic framework particle; MOG, metal-organic gel; MOA, metal-organic aerogel. Figure 1: Schematic representation of the formation of MIL-53(Al) MOF versus AlBDC MOA. MOF, metal-organic framework; MOFP, metal-organic framework particle; MOG, metal-organic gel; MOA, metal-organic aerogel. Full size image Design approach The rational design of supramolecular gels remains a challenge [28] , [29] , [30] . One general process to consider begins with aggregating molecular gelators in one direction to form fibres, which then entangle into a 3D solid network under the aid of supramolecular forces, such as H-bonding, π-π stacking, hydrophobic effects and van der Waals interactions. The formation of MOGs driven by metal–ligand coordination is often difficult because precipitation or crystallization events occur frequently [31] . Nevertheless, various MOGs with coordination polymers acting as discrete or 1D/2D infinite metallogelators have been achieved [27] , [30] , [31] , [32] . To develop highly porous MOAs, the formation of MOGs that display a sponge-like skeletal matrix and not a normal fibrous scaffold is preferred. A convenient approach may be the use of nanoscale MOFPs as subunits in the construction of the 3D gel matrix ( Fig. 1 ). Rigid bridging carboxylate ligands that are suitable for both MOF and MOG assembly [33] , [34] are chosen for this purpose. The cheap and light Al(III) is good for fabrication of the lower density solids of interest to industrial applications at low cost and large scale. The formation of MOFP-based MOGs can be considered to evolve from two main stages. In the early stage of the reaction, the stronger metal–ligand coordination (Al-O bond dissociation energy, Δ H 298 =512 kJ mol −1 ) relative to the metal–solvent interactions causes the metal ions and ligands to assemble into MOF clusters, which then polymerize or aggregate, thus leading to nucleation [24] , [35] , [36] . This process might be dominated by coordination forces, where discrete but periodic MOFPs form as precursors. Over time, as the concentrations of ligands and metal ions decrease, the nucleation of new particles is retarded. In the second stage, the assembly may proceed in two directions. If the reaction conditions favour the crystal growth of the precursors (for example, hydrothermal treatments), the consistent epitaxial growth [37] or oriented attachment [35] induced by surface intension will lead to the crystallization of bulky MOFs (or precipitation due to fast agglomeration). However, if the so-called coordination equilibria [35] are perturbed by other competing interactions, non-crystallographic branching of the MOFPs may occur, thus resulting in mismatched growth or cross-linking and providing the chance for gelation [31] , [38] , [39] . Once the composite MOGs are obtained, the careful removal of the solvents via sub/supercritical CO 2 extraction can leave porous MOAs based on MOFPs ( Fig. 1 ). Various methods have been proposed to control the analogous formation of NMOPs in comparison with nano-MOFPs [4] , [24] , [25] , [26] , [27] , [28] , for example, the addition of initiation solvents [4] or inhibiting agents [28] . However, the gelation behaviours of such nanoscale particles remain largely unexplored [27] . The key step should be to find a balancing condition under which the crystal growth of MOFPs can be surpassed by gelation. We found that moderate heating has a key role in triggering the gelation of proper solvents by MOFPs and not crystallization and/or precipitation. In comparison with other synthetic parameters that influence the gelation process, such as the solvent, concentration, pH, time and sound, heating is seldom recognized to drive a supramolecular system to gel [40] , [41] . In fact, organogels are usually formed via a heating–cooling procedure in which a solution of molecular organogelators is cooled to the glass transition temperature [42] , [43] . For a coordination-driving system, mild heating helps boost the reversibility of the coordination bonding [39] , [43] , making it comparable and competitive with respect to other weak interactions. This creates the prerequisite conditions for the gelation process in the second stage mentioned above ( Fig. 1 ). Under more vigorous conditions (for example, hydrothermal syntheses), coordination will dominate over gelation, which is of benefit to MOF crystallization, because other competitive interactions, such as H-bonding, are significantly easier to diminish and structural transformations are sometimes promoted [44] , [45] , [46] , [47] . Syntheses The preparation of Al-MOGs using a variety of commercially available carboxylic acids was performed. All of the carboxylic acids listed in Supplementary Tables S1 and S2 are capable of inducing Al(III)-gel formation. Typically, the Al-MOGs were prepared through a simple mixing of the metal salt and carboxylic acid solutions ( Supplementary Methods ). At ambient temperature, the mixture remained indefinitely stable, while gelation was observed at properly elevated temperatures. For example, heating the EtOH or DMF-EtOH solutions to 353 K is widely applicable for diverse acids. The gelation state of the materials was evaluated by turning the test tube upside down. The formation of AlBTC and AlBDC gels with different metal-to-ligand ratios and concentrations was tested ( Supplementary Table S3–S6 ), and a detailed gelation process with respect to the reaction temperature was demonstrated for representative AlBDC-3:2-0.15 gels (Al:BDC=3:2, 0.15 mol l −1 based on the ligand, similarly hereafter). The results reveal that temperature is the requisite factor in determining the gelation behaviours, while other factors, such as the metal-to-ligand ratio and concentration, only influence the gelation time and porosity of resulting MOGs. After an adequate aging time, the Al-MOGs were dried by exchanging the pore liquid with CO 2 (l) under subcritical extraction to produce aerogels (Al-MOAs), noting that the direct drying of Al-MOGs usually led to mass losses of solvents/guests entrapped in the gel matrix, which yielded less porous xerogels. Moreover, this gelation approach can be readily generalized to other metal ions to obtain analogous MOFP-based hierarchically porous M-MOGs (M=Fe, Ga and In), as described in the Supplementary Methods . Structural characterization The morphology and microstructure of AlBTC and AlBDC series MOAs were identified using various physical and spectroscopic techniques, including thermogravimetry (TG), scanning electron microscopy (SEM), transmission electron microscopy (TEM), energy dispersive X-ray (EDX), X-ray photoelectron spectra (XPS), infrared (IR), powder X-ray diffraction (PXRD) and NMR analyses ( Supplementary Figs S1–S29 ). Generally, the SEM images show a wormhole-like network skeleton for all of the Al-MOA materials, suggesting that the porous and homogeneous monolithic body of aerogels is made of cross-linked particles rather than normal fibres [24] , [29] , [34] . TEM investigations verify that the agglomerated nanoparticles in aerogels are irregularly interconnected, spanning large void spaces and sustaining the gel matrix ( Fig. 2a ). 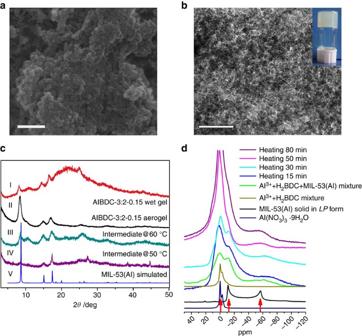Figure 2: Physical characterization of the representative MOAs. (a) SEM of AlBTC-1:1-0.40 (bar width=500 nm). (b) TEM of AlBTC-3:2-0.075 (scale bar, 100 nm; the insert shows digital photograph of gel before subcritical extraction). (c) PXRD patterns of AlBDC-3:2-0.15 wet gel obtained in EtOH at 353 K (I), AlBDC-3:2-0.15 aerogel (II), intermediate obtained from AlBDC-3:2-0.15 reaction systems in EtOH at 333 K (III) and 323 K (IV), and simulation from the single-crystal data of MIL-53(Al) in its LP form (V). (d)27Al MAS NMR spectralex situmonitoring of AlBDC-3:2-0.15 system at different gelation times in comparison with pure Al(NO3)3·9H2O, MIL-53(Al) solid in LP form and their mixtures. Figure 2: Physical characterization of the representative MOAs. ( a ) SEM of AlBTC-1:1-0.40 (bar width=500 nm). ( b ) TEM of AlBTC-3:2-0.075 (scale bar, 100 nm; the insert shows digital photograph of gel before subcritical extraction). ( c ) PXRD patterns of AlBDC-3:2-0.15 wet gel obtained in EtOH at 353 K (I), AlBDC-3:2-0.15 aerogel (II), intermediate obtained from AlBDC-3:2-0.15 reaction systems in EtOH at 333 K (III) and 323 K (IV), and simulation from the single-crystal data of MIL-53(Al) in its LP form (V). ( d ) 27 Al MAS NMR spectral ex situ monitoring of AlBDC-3:2-0.15 system at different gelation times in comparison with pure Al(NO 3 ) 3 ·9H 2 O, MIL-53(Al) solid in LP form and their mixtures. Full size image PXRD was applied to establish the microstructures of the gel materials ( Supplementary Figs S18–S26 ). Representative patterns of the AlBDC-3:2-0.15 aerogel and wet gel are shown in Fig. 2c . The aerogel gives well resolved PXRD patterns with salient peaks that precisely match the simulated patterns of single-crystal MIL-53(Al) in large-pore form (LP form, Supplementary Fig. S27 ) [45] . This implies that the aerogel contains crystalline components of MOF structure, that is, an ordered 3D framework of Al(OH)(BDC) built up from corner-sharing octahedral AlO 4 (OH) 2 chains that are bridged by the benzenedicarboxylate linkers [45] . The broadness of the diffraction peaks indicates that the MOF components in the aerogel are nanoparticles (~10.4 nm, as simulated by the Scherer equation; Supplementary Table S7 ) [28] , which is in agreement with the SEM and TEM observations. The presence of MOPFs in the MOA skeleton is also verified by the solid-state 27 Al and 1 H MAS NMR spectra ( Supplementary Fig. S29 ). The 27 Al NMR spectrum exhibits the superposition of a quadrupolar pattern that is characteristic of the MIL-53(Al) LP form ( δ 27Al =3.4 ppm, C Q =8.4 MHz and η Q =0) ( [45] ). Additionally, the broad peak located at 7.4 ppm is attributed to other coexisting octahedral Al(III)-BDC-solvent motifs. These Al species may bind partially deprotonated H 2 BDC and solvent molecules to form the disordered Al centres and/or Al-hydroxide oligomers [48] , which contribute to gelation by cross-linking the ordered MIL-53 MOFPs and generating the gel scaffold. This notion is further supported by the results of the 1 H MAS NMR analyses. The PXRD pattern and 27 Al NMR of AlBTC-3:2-0.075 MOA also reveal the presence of nano-MOFPs (with sizes ranging from 9.3 to 12.9 nm; Supplementary Table S7 ). However, the structure is not conclusively determined and might contain mixed or unknown phases [49] ( Supplementary Figs S18 and S28 ). Gelation process study To explore when the nano-MOFPs appear along the gelation process, a time- and temperature-dependent ex situ PXRD and 27 Al MAS NMR study was carried out ( Supplementary Figs S30–S33 ). As observed in Fig. 2c , the PXRD patterns of the intermediates obtained for the AlBDC-3:2-0.15 system at 323 and 333 K evidently confirm the appearance of the same crystalline MOFPs as in the final wet gel and aerogel. Moreover, both PXRD and 27 Al NMR suggest that MIL-53 MOFPs form and dominate in the early stage of the gelation process within the present protic medium. However, the transient appearance of and structural transformation from other Al-MOFs may be possible in the initial reaction [44] . The nano-MOFP precursors nucleated in this stage remain almost unchanged in size until the final gelation ( Supplementary Table S8 ); in contrast, time-dependent 27 Al NMR reveals that other disordered Al(III)-BDC-solvent motifs are growing ( Fig. 2d ), which promote the sol–gel transformation by cross-linking the MOFPs and lead to larger irregularly agglomerated nanoparticles. These results support the two-step route proposed above for the construction of MOGs based on MOFP subunits. Further proof for the stepwise formation of MOGs comes from dynamic light scattering (DLS) monitoring of the AlBTC-3:2-0.075 reaction system in EtOH at 353 K ( Supplementary Fig. S34 ). The colloidal sols containing ~12 nm nanoparticles were obtained within 5 min, indicating fast coordination of Al(III) and BTC. This coordination leads to cluster assembly, which is followed by polymerization or aggregation into discrete nano-MOFPs. The MOFP dispersions are stable without a significant increase in colloidal particle size over 10 min, which is consistent with the observed particle sizes of ~11 nm based on the PXRD calculation ( Supplementary Table S7 ). This finding suggests that this period is a nucleation stage, dominated by MOFP precursors formation. Afterward, MOFP agglomeration starts to cause overall particle growth to a size of ~50 nm within 15 min, and speed up growth to ~200 nm in 25 min, falling beyond our DLS limit. The viscosity of the reaction solution continues to increase, and finally, nano-MOFPs gelate solvents throughout the liquid medium to give an open network of MOGs. This period corresponds to the second stage of sol–gel conversion, in which the ordered MOFPs cease to grow larger but the irregularly branching Al(III)-BTC-solvent motifs gradually form to interconnect the MOFP precursors in a long range disordered way. These processes are consistent with the above ex situ PXRD and 27 Al NMR observations, thus verifying the stepwise mechanism of MOG formation from the nano-MOFP colloidal precursors. N 2 sorption and porosity To evaluate the porous properties of the Al-MOAs obtained by subcritical CO 2 (l) extraction of the corresponding Al-MOGs, a series of AlBTC and AlBDC aerogels were subjected to N 2 sorption analyses to determine the surface areas, pore volumes and pore sizes ( Table 1 , Supplementary Tables S9 and S10 ; Fig. 3 , Supplementary Figs S35–S40 ). The N 2 sorption isotherms are between type-I, which is characteristic of microporous materials, and type-IV, which is characteristic of mesoporous materials, showing sheer gas uptake at low pressures and pore condensation with significant adsorption–desorption hysteresis at high pressures. This clearly denotes the coexistence of micro- and mesopores in these Al-MOAs [11] , [12] , [13] . The steep increase in the region of P / P 0 <0.1 is attributed to micropore filling. For the AlBDC-3:2 series MOAs, the Saito-Foley (SF) micropore sizes are narrowly centred at ~0.9 nm, in agreement with the channel size of the MIL-53(Al) crystal in LP form [45] , which further confirms that the MOFPs of MIL-53 contribute to the aerogel microporosity. For the AlBTC-1:1 and AlBTC-3:2 series MOAs, the SF micropore sizes are distributed in a wider range centred at ~1.0 nm ( Supplementary Figs S35 and S36 ), indicating that these MOAs might contain mixed MOF phases. The specific surface areas and mesopore parameters of MOAs can be tuned by changing the reactant concentrations, as observed from the distinguishable sorption behaviours, depending on the reactant concentrations ( Fig. 3 and Supplementary Figs S35 and S36 ). For example, when the concentration of the AlBDC-3:2 gel is 0.05 mol l −1 , the isotherm shows an H2-type hysteresis loop starting at P / P 0 =0.43. The mesoporous volume is ~0.76 cm 3 g −1 , with the mesopores exhibiting a narrow size distribution centred at ~5.4 nm. As the concentration increases to 0.15 mol l −1 , the mesoporous volume significantly increases to ~2.25 cm 3 g −1 , and the pore size becomes larger and wider, centring around ~23.0 nm. The BET surface areas vary up to ~1,324 m 2 g −1 , in accordance with the contributions of the micro- and mesopore volumes, of which the total pore volume is mainly contributed by the mesopores at higher concentration. This is demonstrated by the fact that the hysteresis loops move and condense into higher pressure region (H1-type). At high concentration of 0.2 mol l −1 , the pore sizes show significantly widened distribution at ~87.8 nm, which spans the meso- and macropore sizes. These results are indicative of remarkable influence of concentration on the texture and porosity of MOAs. A similar effect also can be observed for the AlBTC-1:1 and AlBTC-3:2 series ( Supplementary Table S9 ); however, the concentration-pore-size dependency becomes less regular, probably as a result of mixed phases of the MOF particles. Table 1 Porosity properties of selected Al-MOAs based on H 2 BDC and H 3 BTC in ethanol. 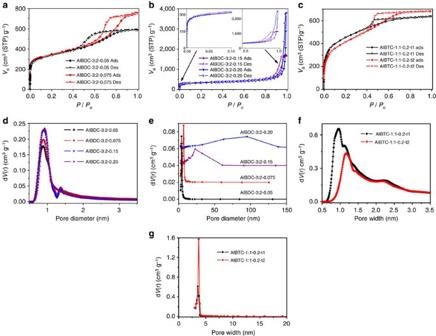Figure 3: Representative N2sorption data. (a,b) The N2adsorption–desorption isotherms of AlBDC-3:2 series MOAs at 77 K (the inserts show enlarged parts of isotherms). (c) The N2adsorption–desorption isotherms of the templated MOAs at 77 K. (d) The SF micropore distribution of the AlBDC-3:2 series MOAs. (e) The BJH pore distribution of the AlBDC-3:2 series MOAs (vertical offsets). (f) The SF micropore distribution of the templated MOAs. (g) The BJH pore distribution of the templated MOAs. Full size table Figure 3: Representative N 2 sorption data. ( a , b ) The N 2 adsorption–desorption isotherms of AlBDC-3:2 series MOAs at 77 K (the inserts show enlarged parts of isotherms). ( c ) The N 2 adsorption–desorption isotherms of the templated MOAs at 77 K. ( d ) The SF micropore distribution of the AlBDC-3:2 series MOAs. ( e ) The BJH pore distribution of the AlBDC-3:2 series MOAs (vertical offsets). ( f ) The SF micropore distribution of the templated MOAs. ( g ) The BJH pore distribution of the templated MOAs. Full size image Template effect In an effort to construct MOAs of more regular mesopores, the supramolecular template strategy has been tested to tune the hierarchical micro/mesoporosity [12] , [13] , [50] . The surfactant cetyltrimethylammonium bromide (CTAB) was used as a structure directing agent, and 1,3,5-trimethylbenzene (TMB) was chosen as an auxiliary agent to swell the CTAB micelles [50] . The AlBTC-1:1 system was selected to prepare the templated MOGs in the presence of CTAB/TMB micelles ( Table 1 and Supplementary Table S9 ). The TEM images show that MOAs AlBTC-1:1-0.2-t1 and AlBTC-1:1-0.2-t2 have more homogeneous wormhole-like mesostructures ( Supplementary Fig. S7 ) compared with the non-templated MOAs, suggesting that the CTAB/TMB micelles can successfully modulate the agglomeration of MOFPs and their gelation behaviour. The N 2 sorption isotherms display a sharp rise of micropore filling in P / P 0 <0.1 region. Additionally, a typical H2-type hysteresis loop can be observed in 0.4< P / P 0 <0.7 region, indicating capillary condensation in the mesopores ( Fig. 3c ). As shown in Supplementary Table S9 , templates effectively regulate the surface areas and mesopore sizes. The BET surface areas of the MOAs significantly increase up to ~1,638 m 2 g −1 , and their mesopore sizes are narrowly distributed at ~3.7 nm (analysed using the BJH algorithm, Fig. 3g ). Increasing the concentration causes a steady increase of the mesopore sizes, but the hysteresis loops show a small change upon reactant and template concentration variation. Density evaluation The density ( ρ ) of MOA materials was calculated using the He and N 2 adsorption data as described in Supplementary Methods ( Supplementary Table S11 ). The easily repeatable sorption data convinced us to estimate the bulk density of the AlBDC-3:2-0.15 MOA as the value of ~0.299 g cm −3 , which is close to the values of the lightest MOF materials reported to date, for example, 0.22 of MOF-200, 0.25 of MOF-210 ( [5] ) and 0.291 of NU-100 ( [6] ). This suggests that the present method used to fabricate hierarchically porous MOAs from gelation of MOFPs may provide a convenient way to achieve ultralight solid materials that incorporate microporous crystalline MOFs into meso-/macroporous aerogel scaffolds. Gas/vapour sorption and separation The high surface area and pore volume of the obtained porous Al-MOAs promote the examination of their H 2 and CO 2 uptake capacity. The H 2 sorption isotherms of MOAs show gradual excess uptake with increasing pressure ( Fig. 4a ; Supplementary Fig. S41 ), and the final storage capacity, for example, AlBTC-1:1-0.8-t2 MOA, reaches 1.52 wt% (the total H 2 uptake is 2.52%) without saturation at 1 bar and 77 K. The pore size variations of different MOAs do not show a significant influence on the H 2 loading, indicating that micropores primarily contribute to H 2 sorption. 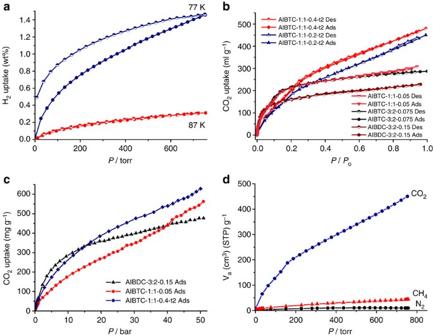Figure 4: Gas uptake and separation data. (a) The H2adsorption–desorption isotherms at 77 and 87 K for the AlBTC-3:2-0.075 MOA. (b) The low-pressure CO2adsorption–desorption isotherms of the various MOAs at 195 K. (c) The high-pressure CO2adsorption–desorption isotherms of the selected MOAs at 298 K. (d) The CO2, CH4and N2adsorption isotherms of AlBTC-1:1-0.2-t2 MOA at 195 K. Figure 4: Gas uptake and separation data. ( a ) The H 2 adsorption–desorption isotherms at 77 and 87 K for the AlBTC-3:2-0.075 MOA. ( b ) The low-pressure CO 2 adsorption–desorption isotherms of the various MOAs at 195 K. ( c ) The high-pressure CO 2 adsorption–desorption isotherms of the selected MOAs at 298 K. ( d ) The CO 2 , CH 4 and N 2 adsorption isotherms of AlBTC-1:1-0.2-t2 MOA at 195 K. Full size image The low-pressure sorption isotherms of CO 2 adsorbed by the MOAs are shown in Fig. 4b and Supplementary Fig. S42 . As representatives, the MOAs AlBTC-1:1-0.05 and AlBTC-3:2-0.075 display CO 2 uptakes of 308 and 287 cm 3 g −1 without saturation at 1 bar and 195 K, corresponding to 61 and 56 wt%, respectively. Interestingly, the templated MOAs, with increasingly ordered mesoporosity, show significantly higher CO 2 adsorption capacity, that is, up to 480 cm 3 g −1 (21.4 mmol g −1 , 94 wt%). A similar tendency can be observed for the high-pressure CO 2 uptake at 298 K up to 50 bar ( Fig. 4c ). All isotherms were not saturated, and a high CO 2 uptake of 627 mg g −1 (14.3 mmol g −1 , 63 wt%) was achieved by AlBTC-1:1-0.4-t2 MOA at 298 K. This suggests that the narrowly ordered mesoporosity may contribute to the larger CO 2 uptake, offering a CO 2 loading capacity among the highest values of MOFs, such as MOF-177, 205, 200, 210 and NU-100 under similar conditions at both high and low temperatures [5] , [6] , [51] . The enhanced CO 2 capture of the hierarchically porous MOAs can be attributed to the strong physisorption of CO 2 onto the unsaturated metal sites on the surface of the inter-crystallite mesopores, which was examined and demonstrated by the in situ IR spectroscopy study of CO 2 and pyridine adsorption ( Supplementary Figs S43 and S44 ). To evaluate the gas separation ability of the porous MOAs, the templated MOA AlBTC-1:1-0.2-t2 was selected for study: its gas-uptake behaviours for CH 4 , N 2 and CO 2 at 195 K were measured. The sorption isotherms reveal little CH 4 and N 2 adsorption but an uptake of 450 cm 3 g −1 (88.4 wt%) for CO 2 ( Fig. 4d ). The calculated Henry CO 2 /N 2 and CO 2 /CH 4 separation selectivities are 23.2 and 3.05 ( Supplementary Table S12 , Supplementary Fig. S45 ), respectively. Such separation selectivity, that is, favouring CO 2 over other gases, implies a potential application in the separation of industrial gases for the presented readily fabricated porous MOAs. The vapour sorption properties were also tested for the AlBDC MOAs by selecting chemically different adsorbates, that is, non-polar aromatic benzene, linear n -hexane and polar methanol ( Supplementary Figs S46–S48 ). Generally, all sorptions onto aerogels are reversible, and the isotherms are close to type IV but show steep initial uptakes and significant hysteresis loops in a wide P / P 0 range after the micropore filling. Such stepwise adsorption and the remarkable hysteresis loop obviously can be attributed to the unique features of the hierarchical MOAs, which combined the mesoporous nature with the flexible nature that is characteristic of microporous MIL-53(Al) ( [45] , [52] ). With respect to the adsorption capabilities, the aerogels adsorb benzene up to 247 cm 3 g −1 (86 wt%), n -hexane up to 122 cm 3 g −1 (47 wt%), and methanol up to 672 cm 3 g −1 (96 wt%). Dye uptake To verify the accessibility of the MOAs for bulky molecule transportation, the aerogel AlBDC-3:2-0.15 was selected as a represented for the dye uptake test. The adsorption of congo red (CR) and brilliant blue R-250 (BBR-250) dyes was studied using UV–vis spectroscopy ( Fig. 5a ). The porous MOA displays a fast uptake of these dye molecules. Upon adsorption equilibrium, the high adsorbing capacities reach 633.4 and 621.3 mg g −1 for CR and BBR-250, respectively. This simply demonstrates that the mesopores of the MOAs are readily accessible to bulky organic molecules, which, in turn, may be able to facilitate interactions between the guests and micropores to enhance, for example, catalytic activity by nanoscale MOFPs. 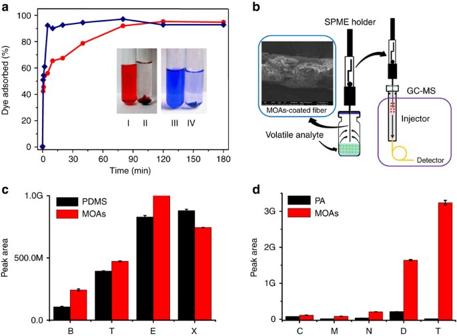Figure 5: Dye uptake and SPEM data. (a) The kinetic curves of the AlBDC-3:2-0.15 MOA (7.5 mg) in 50 ml of dyes solution (100 mg l−1) for congo red (circle) and brilliant blue R-250 (square). The inserts show pictures of the dye-polluted water (I, III) before and (II, IV) after dye adsorption. (b) A schematic demonstration of the SPME analyses of a volatile analyte using the MOA-coated fibres (SEM image). (c) The extraction contrast profiles with AlBTC-3:2-0.05 MOA-coated and PDMS fibres for 1 ppm BTEX compounds. (d) The extraction contrast profiles with AlBTC-3:2-0.05 MOA-coated and PA fibres for 1 ppm phenols. The conditions for BTEX: extraction temperature, 298 K; extraction time, 10 min (stirring); desorption time, 0.5 min. PDMS, polydimethylsiloxane; B, benzene; T, toluene; E, ethylbenzene; X, xylene. Conditions for phenols: extraction temperature, 298 K; extraction time, 20 min (stirring); desorption time, 1 min. PA, polyacrylate; C, 2-chlorophenol; M, 4-methylphenol; N, 2-nitrophenol; D, 2,4-dichlorophenol; T, 2,4,6-trichlorophenol. Figure 5: Dye uptake and SPEM data. ( a ) The kinetic curves of the AlBDC-3:2-0.15 MOA (7.5 mg) in 50 ml of dyes solution (100 mg l −1 ) for congo red (circle) and brilliant blue R-250 (square). The inserts show pictures of the dye-polluted water (I, III) before and (II, IV) after dye adsorption. ( b ) A schematic demonstration of the SPME analyses of a volatile analyte using the MOA-coated fibres (SEM image). ( c ) The extraction contrast profiles with AlBTC-3:2-0.05 MOA-coated and PDMS fibres for 1 ppm BTEX compounds. ( d ) The extraction contrast profiles with AlBTC-3:2-0.05 MOA-coated and PA fibres for 1 ppm phenols. The conditions for BTEX: extraction temperature, 298 K; extraction time, 10 min (stirring); desorption time, 0.5 min. PDMS, polydimethylsiloxane; B, benzene; T, toluene; E, ethylbenzene; X, xylene. Conditions for phenols: extraction temperature, 298 K; extraction time, 20 min (stirring); desorption time, 1 min. PA, polyacrylate; C, 2-chlorophenol; M, 4-methylphenol; N, 2-nitrophenol; D, 2,4-dichlorophenol; T, 2,4,6-trichlorophenol. Full size image SPME analyses To test the potential applications of the present hierarchically porous MOAs with respect to their features of facile preparation and immobilization in a readily handled shape and monolith, we selected AlBTC-3:2-0.05 MOA as the coating adsorbent, used to prepare fibres for the solid-phase microextraction [53] (SPME, Fig. 5b and Supplementary Fig. S49 ). A series of experiments were performed to evaluate the performance of the MOA adsorbents for SPME analyses, including BTEX and phenolic compounds. To extract four non-polar compounds (BTEX) using headspace-SPME (HS-SPME), the MOA-coated fibres shows generally higher extraction efficiency than the commercial 100-μm PDMS fibres ( Fig. 5c ). For five polar compounds (phenols), the aerogel fibres exhibit both higher extraction efficiency and excellent selectivity, for example, up to 228 times for 2,4,6-trichlorophenol, in comparison with the commercial 85-μm PA fibres ( Fig. 5d ). Additionally, the extraction time required to reach equilibrium and the desorption time necessary to activate the fibres are short. Further, the selective extractions with respect to BTEX and phenols are obviously superior to the commercial fibres. The repeated measurements of both the BTEX and phenol SPME analyses confirm that the MOA-coated fibres retain their effectiveness over several runs ( Supplementary Tables S13–S16 ). We have demonstrated a general pathway for the production of a variety of hierarchically porous Al(III)-MOAs, based on the stepwise gelation of MOF nanoparticles. These materials feature the desirable physical properties of aerogels, exhibiting high surface area, large pore volume and low density, while also integrating the ordered microporosity of crystalline MOFs into overall gel matrix. The MOA materials can be prepared at the gram scale and are easy to handle. The key factor that induces the sol–gel transition is the selection of an appropriate gelation temperature. The mesoporous levels of the aerogels can be readily modified by varying the reactant concentration and are well regulated by supramolecular templates, providing an alternative synthetic approach to meso-MOF materials with hierarchical porosity. Their micropores and mesopores are accessible to various guest molecules, as revealed by gas/vapour sorption and bulky dye uptake experiments. The aerogels’ potential applications as SPME fibre-coating materials were tested, suggesting that the porous MOAs exhibit good extraction and enrichment performance and high molecular diffusivity in the SPME analyses and may be promising in SPME fibre coatings with high capacity, selectivity and sensitivity. Additionally, owing to their structural features, which incorporate MOF diversification and MOG mass immobilization, both convenient modification and structural tuning are possible with respect to specific functionality, such as gas storage, separation, membrane, catalysis, sensing and drug delivery. Materials and measurements All chemicals and solvents are commercially available and were used as received. The dry solvents were treated on a MB-SPS-5 solvent system. The physical and spectroscopic measurements, including TG, SEM, TEM, EDX, XPS, IR, UV–vis, PXRD, DLS, and solid-state MAS NMR analyses, are summarized in the Supplementary Methods . The gelation test with different ligands and metal ions, characterization of the MOG and MOA materials, the study of the gelation process, the N 2 sorption and porosity analyses, the density calculations, the gas/vapour sorption and separation analyses, and the SPME analyses are described in detail in the Supplementary Methods . Typical synthetic procedure represented by AlBTC-1:1-0.2 system H 3 BTC (42.4 mg, 0.2 mmol) and Al(NO 3 ) 3 ·9H 2 O (75.0 mg, 0.2 mmol) were each dissolved in EtOH (0.5 ml), and the two solutions were rapidly mixed together. The resulting homogeneous solution was then allowed to stand at 353 K for gelation in a closed container. A MOG was obtained after ~30 min. After gelation, the wet gel was aged for 2 days at 353 K. Subsequently, the wet gel was subjected to solvent exchange with ethanol for 1 day using a Soxhlet extractor. The as-prepared gel was placed into a high-pressure Soxhlet extractor (0.75 l). The solvent in the wet gel was extracted with liquid CO 2 (265–270 g) for 20 h, and the extraction temperature was maintained at 308 K. The MOA product was obtained after depressurizing the stainless-steel autoclave slowly at room temperature for ~2–3 h. The detailed reaction parameters and product information for the various gel materials are listed in Supplementary Tables S1–S6 . How to cite this article: Li, L. et al . A synthetic route to ultralight hierarchically micro/mesoporous Al(III)-carboxylate metal-organic aerogels. Nat. Commun. 4:1774 doi: 10.1038/ncomms2757 (2013).